Asymmetric total synthesis of (−)-lingzhiol via a Rh-catalysed [3+2] cycloaddition The development of efficient reactions for the one-pot construction of bicyclic ring systems bearing two quaternary carbon centres at their bridgehead positions represents a significant challenge to synthetic chemistry. The development of new methods capable of overcoming this challenge is highly desirable, because this motif can be found in a wide range of natural products with significant biological activities. Herein, we report an efficient [3+2] cycloaddition reaction between an enal and an alleno rhodium species, which was generated in situ from the corresponding enynol via a retro metal-propargylation reaction, to give [3.3.0] and [3.4.0] bicyclic systems bearing two quaternary atoms at their bridgehead positions. The developed chemistry has been successfully applied to the asymmetric total synthesis of natural product (−)-lingzhiol ( 4 ) for the first time in 17 steps. A wide variety of intriguing natural products with five-membered [3.3.0] and [4.3.0] carbobicyclic ring systems and two vicinal stereogenic quaternary carbon centres at the ring junction have been identified to exhibit significant biological activities that could potentially be used to develop new drugs [1] , [2] , [3] , [4] , [5] , [6] . Subergorgic acid ( 1 in Fig. 1a ), isolated from the Pacific gorgonian coral Subergorgia subeross , showed cardiotoxic activity [1] . Crinipellin A ( 2 ), isolated from the fungus Crinipellis stipitaria (Agaricales), has been reported to exhibit potent antibiotic activity [2] . Retigeranic acid ( 3 ) is a representative member of the sesterterpenoid family of compounds and exhibits a broad range of biological activities [3] , [4] , [5] , [6] , [7] . Although compounds of this type are well known to elicit a variety of interesting biological responses, efficient methods for their construction are scarce. New synthetic strategies and methodologies are therefore required to provide facile access to these natural products and their analogues, to allow for the development of new therapeutic agents and drugs. 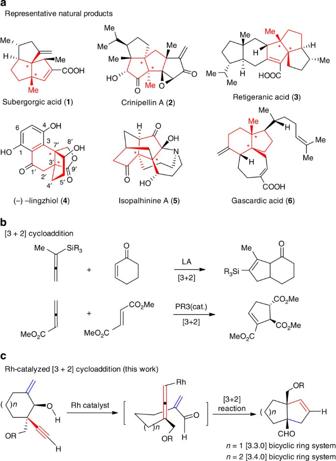Figure 1: Representative natural products containing five-membered carbocycles and their synthetic methods. (a) Selected biologically active natural products bearing bridgehead functionalized [3.3.0] fused rings and [3.4.0] fused rings. (b) Lewis acid-promoted and phosphine-catalysed [3+2] cycloaddition of allenoates to construct five-membered carbocycles. (c) Our strategy to access both [3.3.0] and [4.3.0] bicyclic ring systems via Rh-catalysed [3+2] cycloaddition. Figure 1: Representative natural products containing five-membered carbocycles and their synthetic methods. ( a ) Selected biologically active natural products bearing bridgehead functionalized [3.3.0] fused rings and [3.4.0] fused rings. ( b ) Lewis acid-promoted and phosphine-catalysed [3+2] cycloaddition of allenoates to construct five-membered carbocycles. ( c ) Our strategy to access both [3.3.0] and [4.3.0] bicyclic ring systems via Rh-catalysed [3+2] cycloaddition. Full size image The construction of vicinal quaternary carbon centres, however, represents a significant challenge in natural-product synthesis [8] . Despite significant progress in this area during the last two decades towards the stereoselective synthesis of vicinal quaternary carbon centres [9] , [10] , [11] , [12] , [13] , [14] , [15] , [16] , there are currently no efficient reactions available for the enantioselective construction of [3.3.0] and [4.3.0] bicyclic ring systems [17] , [18] bearing two quaternary carbon centres at their bridgehead positions. This lack of suitable synthetic methodologies has therefore limited the in-depth exploitation of the biological and pharmaceutical value of these natural products. Five-membered carbocycles can be constructed according to reactions between 3-C and 2-C units [19] , [20] . Danheiser and Becker [21] reported the use of an allene as a three-carbon synthon in their [3+2] cycloaddition reaction of Si-substituted allenes ( Fig. 1b ). In a separate study, Lu et al. [22] , [23] reported the development of a phosphine catalysed [3+2] cycloaddition reaction. Recently, phosphine-catalysed regio- and enantio-selective [3+2] cycloadditions of allenoates with electron-deficient olefins and imines—a process that provided efficient access to a variety of synthetically useful carbo- and hetereocycles—have received considerable research interest, and significant progresses have been elegantly demonstrated by different groups [24] , [25] , [26] , [27] , [28] , [29] , [30] , [31] , [32] , [33] . Despite the above impressive achievements, there is an urgent need for the development of efficient [3+2] cycloaddition reaction to enable the direct and stereoselective syntheses of [3.3.0] and [4.3.0] bicyclic ring systems bearing two quaternary carbon centres at their bridgehead positions. As a useful nucleophile, allenyl metal species can react with a wide variety of electrophiles [34] , [35] , [36] and, consequently, these adducts have been applied to the syntheses of a broad range of structurally diverse compounds [37] , [38] , [39] . However, the use of allenyl rhodium species in organic synthesis remains scarce [40] , [41] , [42] . With this in mind, and as part of our ongoing work towards the development of efficient methods for the total synthesis of natural products, we investigated the use allenyl rhodium species as three-carbon synthons in organic synthesis. It was envisaged that the use of an α,β-unsaturated aldehyde linked to an allenyl rhodium moiety could be used for an intramolecular [3+2] cycloaddition reaction, which would allow for the formation of a cyclopentane ring [43] , [44] . Herein, we report the development of a new [3+2] cycloaddition reaction between an enal and an alleno rhodium species, which was generated in situ by the Rh(I)-mediated retro-propargylation of homo-propargyl alcohol [45] , to give [3.3.0] and [4.3.0] bicyclic ring systems bearing two quaternary carbon centres at the bridgehead positions ( Fig. 1c ). Notably, the use of chiral starting materials in this reaction led to the unprecedented synthesis of enantiomerically pure [3.3.0] bicyclic products, representing a significant development in terms of the application of this reaction to the total synthesis of naturally occurring biologically active chiral molecules. Furthermore, this newly developed reaction has been successfully applied to the total synthesis of natural product lingzhiol, which is reported to be an important agent for the study and treatment of diabetic nephropathy [4] . Optimization of the reaction conditions During the course of this study, compound 7a (entry 1 in Table 1 ), which contained a homo-propargyl alcohol and a terminal alkene, was converted to 7b in 23% yield as a single diastereoisomer in the presence of [RhCl(cod)] 2 (5 mol%) under a balloon pressure of CO. The structure of 7a was confirmed by X-ray crystallographic analysis of its precursor diol, and this observation inspired us to investigate this reaction in greater detail. Table 1 Catalyst screening and reaction optimization conditions. Full size table Initial optimization of the reaction conditions have been performed on studying the effects of various reaction parameters on the outcome of the reaction, including the type of rhodium catalyst, the solvent and the temperature. Of the different rhodium catalysts and solvents tested, [RhCl(CO) 2 ] 2 (refs 46 , 47 , 48 ) in ClCH 2 CH 2 Cl was found to be optimal. To demonstrate the catalytic role of the rhodium catalyst, the annulation reaction of 7a was conducted in the absence of [RhCl(CO) 2 ] 2 ; as a result, no annulated product 7b was observed, indicating that the rhodium catalyst was essential to the success of the reaction. We then carried out the reaction below 80 °C and the reaction became sluggish, which resulted in lower yields of the annulated product 7b . The results of these screening experiments were combined into a single optimized procedure involving the use of a catalytic amount of [RhCl(CO) 2 ] 2 (5 mol%) at a temperature of 85 °C under a positive pressure of CO (balloon) in ClCH 2 CH 2 Cl, which gave the annulated 7b in an isolated yield of 87% (entry 7 in Table 1 ). It is noteworthy that these reactions had to be conducted under an atmosphere of CO. When the reaction was conducted in the absence of CO, the desired product 7b was formed in a reduced yield of only 45% (entry 8 in Table 1 ). To determine whether the observed low yield occurred as a consequence of a Rh-catalysed decarbonylation [49] reaction, we monitored the reaction by high-resolution mass spectroscopy, although the results of this analysis failed to identify the formation of a decarbonylative species during the course of the reaction ( Supplementary Fig. 80 ). Based on these results, it was proposed that under an atmosphere of CO, the decomposition of [RhCl(CO) 2 ] 2 catalyst was in part prohibited, thus facilitating the conversion from 7a to 7b . 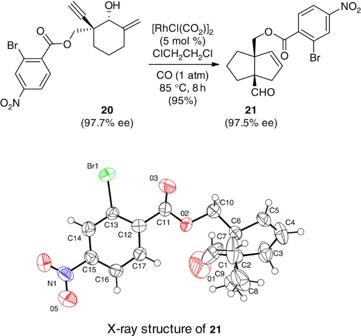Figure 2: Chirality transfer. Enantiomerically enriched substrate20underwent Rh-catalysed [3+2] cycloaddition to yield enantiomerically enriched product21. Substrate scope To assess the scope and generality of the optimized reaction conditions, we prepared enynols 8a – 14a in their racemic forms and investigated their annulation under the conditions listed in Table 2 . Substrates 8a – 11a , bearing an ether, ester or carboxylate substituent ( Table 2 , entries 2–4), can give the corresponding annulated products 8b – 11b in good-to-excellent yields (68–98%). Furthermore, the alkyne moiety of the substrate could be substituted with an aromatic group, which demonstrated that moderate reaction yields could be achieved in most cases ( Table 2 , entry 6). However, when the substrates bear a bromine substituent at the terminal alkyne position (entry 5, 12a ), or two methyl groups at the exocyclic methylene positions (entry 7, 14a ), the yields for the annulation are relatively low due to the substrate decomposition under the standard conditions. Table 2 Synthesis of the [3,3,0]-bicyclic scaffolds. Full size table The annulation reaction is also compatible with the presence of a bromine substituent at the terminal alkyne position, although the corresponding [3+2] product 12b was isolated in low yield due to the stability problems. The substitution of the exocyclic methylene group with two methyl groups was also well tolerated under the optimized conditions ( Table 2 , entry 7), with the annulated product 14b being isolated in a yield of 43%. This particular example highlights the potential value of applying our method as a strategy for the construction of up to three vicinal quaternary carbon centres. The structure of 10b was confirmed by X-ray crystallographic analysis. 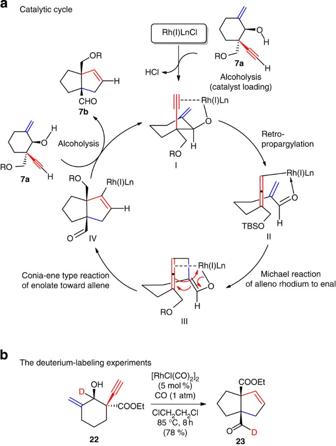Figure 3: Proposed Rh-catalysed reaction cycle and deuterium-labelling experiments. (a) The possible mechanism involves the sequential Rh-catalysed retro-propargylation/intramolecular Michael addition/Conia-ene-type reaction/alcoholysis. (b) The deuterium-labelling experiments indicate that the aldehyde is generated via a Rh-mediated C–C bond cleavage reaction. We also investigated the application of our newly developed reaction as a general method for the construction of [4,3,0] ring systems ( Table 3 ). Enynols 15a – 19a were prepared and subjected to the optimized reaction conditions to afford the corresponding products 15b–19b in good-to-acceptable yields, bearing two syn -configured vicinal quaternary stereocentres. These results highlight the robust nature of our method as a general strategy for the construction of ring systems of different sizes. The structure of 16b was confirmed by X-ray crystallographic analysis. Table 3 Syntheses of the [3,4,0]-bicyclic scaffolds. Full size table It is particularly important that optically active molecules can be readily and reliably generated during the course of a total synthesis of natural product, because the optical properties of a molecule can have a significant impact on its biological activities. With this in mind, we evaluated the ability of optical enynols to undergo a stereospecific [3+2] cycloaddition reaction without affecting their original enantiomeric excess (ee). The chiral enynol ester 20 (97.7% ee, Fig. 2 ) was readily synthesized from the corresponding chiral enynol via a coupling reaction with 2-bromo-4-nitrobenzoic acid. The application of the optimized annulation conditions to 20 resulted in the formation of the cycloaddition product 21 (97.5% ee) in 95% yield ( Supplementary Figs 77 and 78 ). The stereochemistry of 21 was confirmed through X-ray crystallography. These results indicated that this [3+2] cycloaddition reaction occurred in a stereospecific manner, and that the chirality of the substrate was effectively transferred to the product. Figure 2: Chirality transfer. Enantiomerically enriched substrate 20 underwent Rh-catalysed [3+2] cycloaddition to yield enantiomerically enriched product 21 . Full size image Mechanism investigation Although the mechanism of this reaction is not completely elucidated, we proposed a mechanism to account for the stereochemical outcome of the reaction ( Fig. 3a ). It was envisaged that [RhCl(CO) 2 ] 2 would react with compound 7a to afford complex I (refs 50 , 51 ), which would undergo a Rh(I)-mediated retro-propargylation of the homopropargyl alcohol to afford complex II ( Fig. 3a ). Figure 3: Proposed Rh-catalysed reaction cycle and deuterium-labelling experiments. ( a ) The possible mechanism involves the sequential Rh-catalysed retro-propargylation/intramolecular Michael addition/Conia-ene-type reaction/alcoholysis. ( b ) The deuterium-labelling experiments indicate that the aldehyde is generated via a Rh-mediated C–C bond cleavage reaction. Full size image Complex II would then undergo the intramolecular Michael addition [52] , [53] , [54] , [55] , [56] of the allenyl rhodium to the enal, to give the allenyl rhodium species III bearing an enolate moiety and a Rh-coordinate allene moiety. The transformation of III to IV can be interpreted as a Conia-ene [57] -type reaction between the Rhoda-enolate species and the allene. Finally, protonolysis [58] , [59] , [60] of complex IV with 7a would give product 7b , which contains a [3.3.0] bicyclic ring moiety, together with the regeneration of complex I , which would allow for the completion of the catalytic cycle. To support our proposed reaction mechanism, the deuterated enynol 22 was prepared as a probe to confirm that the Rh(I)-catalysed retro-β-carbon elimination reaction was the key step in our catalytic cycle ( Fig. 3a ). The annulation of 22 under the optimized reaction conditions gave the desired product 23 in 78% yield with the retention of deuterium ( Fig. 3b ). This result indicated that the aldehyde substituent at the C1 position was generated via a Rh-mediated C–C bond cleavage reaction, rather than the oxidation of the corresponding alcohol. Computational study To further support our proposed reaction mechanism, density functional theory method M11-L, recently proposed by Peverati and Truhlar [61] , is employed to elucidate the mechanism of Rh-catalysed reaction cycle ( Supplementary Tables 1 and 2 ). The free-energy profile, shown in Fig. 4 , indicates that intramolecular retro metal propargylation from CP1 to CP2 occurs via a concerted transition state TS1 with an activation-free energy of 16.9 kcal mol −1 . The allene–rhodium complex CP2 then forms reversibly, with the chirality of the allene being determined by the α-carbon of the alkyne moiety in CP1 . In CP2 , the enone moiety is activated by rhodium (similar to the Lewis acid activation of enones), because the oxygen atom in the enone moiety coordinates to the rhodium atom. The second step, which is the rate limit, in this process is a relatively facile Michael-type addition of alleno–rhodium to the activated enone via TS2 , with an activation-free energy of 24.4 kcal mol −1 . This Michael-type addition reaction affords intermediate CP3 , which contains an enolate moiety and an allene moiety. 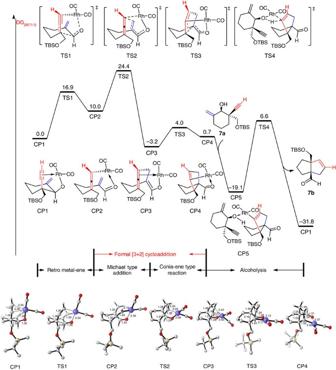Figure 4: Density functional theory calculations. Free-energy profiles and geometric information for catalytic cycle of rhodium-catalysed synthesis of bicyclo[3.3.0]octane7b. Figure 4: Density functional theory calculations. Free-energy profiles and geometric information for catalytic cycle of rhodium-catalysed synthesis of bicyclo[3.3.0]octane 7b . Full size image The allene moiety in CP3 is activated by its coordination to the rhodium centre. The subsequent reaction is alkylation of the enolate by the activated allene via a Conia-ene-type reaction. This alkylation step via TS3 is facile and gives the formal intramolecular [3+2] cycloadduct CP4 , with an activation-free energy of 7.2 kcal mol −1 . The last step is demetalation by the alcohol moiety of the substrate, which begins with ligand exchange between CP4 and the starting material 7a to give CP5 . Next, the C–Rh bond in complex CP5 is protonated via four-membered-ring transition state TS4 (ref. 62 ). Following the release of product 7b , the active intermediate CP1 is regenerated irreversibly to complete the catalytic cycle. This mechanism also well explains how the chirality in the starting molecule can be transferred to the final [3+2] cycloadduct. Total synthesis of (−)-lingzhiol To demonstrate the utility of our newly developed methodology, we applied the annulation reaction in the asymmetric total synthesis of (−)-lingzhiol ( 4 ) [4] . As a pair of rotary door-shaped meroterpenoidal enantiomers, (−)-lingzhiol ( 4 ) and its enantiomer (+)-lingzhiol were isolated from Ganoderma lucidum by Hou and colleagues [4] , who had to use 80 kg of G. lucidum to obtain 25 mg of both pure (−)-lingzhiol and (+)-lingzhiol. G. lucidum is a well-known mushroom that is used extensively in Asia as a super-grade medicine. Biological studies of the chemicals contained in this mushroom have indicated that both of the enantiomers of lingzhiols show potent and selective inhibitory activity towards the phosphorylation of Smad3 in transforming growth factor-β1-induced rat renal proximal tubular cells and activate Nrf2/Keap1 in mesangial cells under diabetic conditions [4] . In light of the important biological activities of lingzhiol-type compounds and their potential application as lead compound for the development of therapeutic agents against chronic kidney disease, there is an urgent need for the development of a synthetic method capable of providing facile access to these materials to allow for detailed studies of their structure–activity relationship. From a chemical perspective, (−)-lingzhiol ( 4 ) represents a formidable challenge for total synthesis. (−)-Lingzhiol ( 4 ) possesses an intricate structure, which is decorated with two syn -configured vicinal quaternary carbon centres at the bridgehead carbons. This compound is also composed of a highly compact carbobicyclo[4.3.0]nonane core, which is known as a dihydroquinone-fused propellane. The development of an efficient synthesis for (−)-lingzhiol ( 4 ) that proceeds with good stereoselectivity would allow for the preparation of the natural product as well as its analogues in large-enough quantities to facilitate an adequate evaluation of their biological activities. Our synthetic strategy was devised to provide rapid access to asymmetric synthesis of (−)-lingzhiol ( 4 ) and to address the synthetic issues associated with the construction of the highly compact carbobicyclo[4.3.0]nonane core belonging to this structural class. It was envisaged that our newly developed Rh-catalysed intramolecular [3+2] cycloaddition reaction could be used for the stereoselective formation of the carbobicyclo[4.3.0]nonane core of (−)-lingzhiol ( 4 ), because this reaction would allow for the installation of the two bridgehead and syn -configured vicinal quaternary carbon centres in a single step. Our retrosynthetic analysis of (−)-lingzhiol ( 4 ) is shown in Scheme 3. It was envisaged that the application of allylic oxidation, benzylic oxidation and demethoxylation reactions would allow for the successful elaboration and conversion of chiral lactone 24 into the final product (−)-lingzhiol ( 4 ). Lactone 24 could be synthesized directly from the tricyclic precursor aldehyde 25 via a reductive lactonization reaction. The disconnections of the C3′–C7′ and C4′–C6′ bonds of 25 led to the homopropargyl alcohol 26 , which could undergo our newly developed Rh-catalysed intramolecular [3+2] cycloaddition reaction to form the tricyclic core of 25 in a diastereoselective manner. The chiral homopropargyl alcohol 26 could be prepared from enone 27 via sequential asymmetric ketone reduction with ( R )-CBS/BH 3 (ref. 63 ), carboxylation and alkynylation [64] reactions. In this way, our retrosynthetic analysis was traced back to the preparation of enone 27 , which could be made from commercially available 5,8-dimethoxy-3,4-dihydronaphthalen-1(2 H )-one ( 28 ) ( Fig. 5 ). 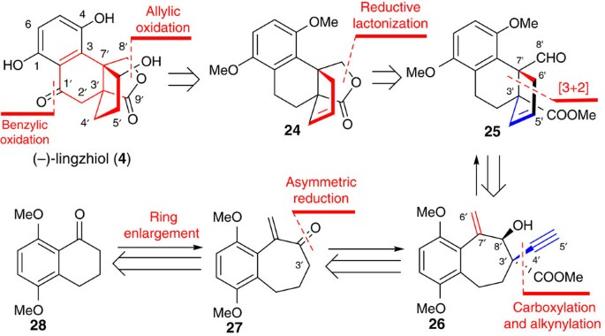Figure 5: Retrosynthetic analysis of (−)-lingzhiol. The current Rh-catalysed [3+2] cycloaddition was used as a key step to construct the [4.3.0]-bicyclic ring moiety in (−)-lingzhiol. Figure 5: Retrosynthetic analysis of (−)-lingzhiol. The current Rh-catalysed [3+2] cycloaddition was used as a key step to construct the [4.3.0]-bicyclic ring moiety in (−)-lingzhiol. Full size image Our total synthesis of (−)-lingzhiol ( 4 ) began with the asymmetric preparation of the homo-propargyl alcohol 26 ( Fig. 6 ). Treatment of commercially available 5,8-dimethoxy- 3,4-dihydronaphthalen-1(2 H )-one ( 28 ) with a mixture of Ph 3 PCH 3 Br and potassium bis(trimethylsilyl)amide (KHMDS) in tetrahydrofuran (THF) resulted in the formation of the expected olefin in 98% yield, which was subsequently reacted with Koser’s reagent [65] in the presence of p -TSA in MeCN to give the benzoannulenone 29 in 95% yield via a ring-expansion reaction. Compound 29 was initially reacted with formyl aldehyde under a variety of different conditions. Unfortunately, however, the desired aldol reaction did not occur under these conditions, presumably because of the poor reactivity of formaldehyde. Alternatively, starting from Eschenmoser’s salt, which was prepared by the reaction of formaldehyde with Et 2 NH·HCl/Et 2 NH, the aldol reaction with ketone 29 in 1,4-dioxone at 105 °C furnished the expected enone 27 in almost quantitative yield, which then subjected to an asymmetric reduction with ( R )-CBS/BH 3 to afford the chiral allylic alcohol 30 in 91% yield with 94% ee. 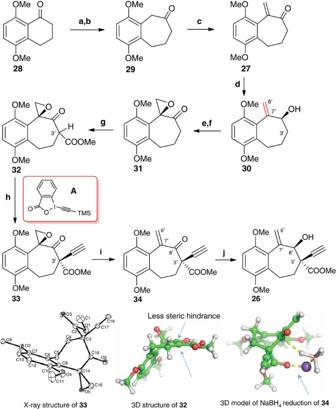Figure 6: Synthetic pathways for the construction of intermediate26. (a) PPh3CH3Br, THF, KHMDS 0 °C to 25 °C, 98%; (b) PhI(OAc)2, p-TSA, MeCN, 0 °C, 95%; (c) Et3N·HCl, Et2NH, (CH2O)n, 1,4-dioxone, 105 °C, 98%; (d) (R)-CBS, BH3, THF, −20 °C, 91%, 92% ee; (e) meta-chloroperoxybenzoic acid (m-CPBA), NaHPO4, PhH, 25 °C; (f) Dess–Martin periodinane, NaHCO3, DCM, 25 °C, 81% for two steps; (g) LiHMDS, NCCOOMe, THF, −78 °C; (h) tetra-n-butylammonium fluoride,A, THF, −30 °C, 62% for two steps; (i) NaI, MeCN, CF3COOH, 0 °C, 92%; (j) NaBH4, CeCl3·7H2O, EtOH, 0 °C, 63%. KHMDS: Potassium bis(trimethylsilyl)amide. Figure 6: Synthetic pathways for the construction of intermediate 26 . ( a ) PPh 3 CH 3 Br, THF, KHMDS 0 °C to 25 °C, 98%; ( b ) PhI(OAc) 2 , p-TSA, MeCN, 0 °C, 95%; ( c ) Et 3 N·HCl, Et 2 NH, (CH 2 O) n , 1,4-dioxone, 105 °C, 98%; ( d ) (R)-CBS, BH 3 , THF, −20 °C, 91%, 92% ee; ( e ) meta-chloroperoxybenzoic acid ( m -CPBA), NaHPO 4 , PhH, 25 °C; ( f ) Dess–Martin periodinane, NaHCO 3 , DCM, 25 °C, 81% for two steps; ( g ) LiHMDS, NCCOOMe, THF, −78 °C; ( h ) tetra-n-butylammonium fluoride, A , THF, −30 °C, 62% for two steps; ( i ) NaI, MeCN, CF 3 COOH, 0 °C, 92%; ( j ) NaBH 4 , CeCl 3 ·7H 2 O, EtOH, 0 °C, 63%. KHMDS: Potassium bis(trimethylsilyl)amide. Full size image With the chiral allylic alcohol 30 in hand, we turned our attention towards its elaboration to the key intermediate 26 . To this end, allylic alcohol 30 was first subjected to a substrate-controlled asymmetric epoxidation by reaction with meta-chloroperoxybenzoic acid to afford an epoxide, which was then oxidized to ketone 31 in 81% yield in two steps by the treatment with Dess–Martin periodinane in the presence of NaHCO 3 in CH 2 Cl 2 . To install the functional groups at its C3′ position, ketone 31 was reacted with LiHMDS in THF at −78 °C, followed by reaction with methyl carbonocyanidate to give the β-ketoester 32 as a pair of ketone-enol isomers. Compound 32 was found to be unstable and was therefore immediately reacted with Waser’s reagent [66] in the presence of tetra- n -butylammonium fluoride in THF at −30 °C to give compound 33 in 62% yield in two steps, together with 10% of its diastereisomer. The stereochemistry of 33 was confirmed through X-ray crystallography and the observed diastereoselectivity presumably occurred as a consequence of the less steric hindrance of the top face of 32 (see the three-dimensional (3D) structure of 32 in Fig. 6 ). Thus, the treatment of compound 33 with NaI in the presence of CF 3 COOH in MeCN provided ketoester 34 in 92% yield. Finally, the Luche reduction [67] of ketoester 34 with NaBH 4 in the presence of CeCl 3 ·7H 2 O in ethanol at 0 °C gave the homo-propargyl alcohol 26 in 63% yield as a single isomer. To account for the observed diastereoselectivity, we proposed that the ester group of 34 could coordinate with NaBH 4 in such a way as to facilitate the delivery of the hydride to the ketone from its bottom face (see 3D model of complex 34 in Fig. 6 ). We then proceeded to evaluate our newly developed Rh-catalysed [3+2] cycloaddition reaction with the homo-propargyl alcohol 26 for the stereoselective construction of the critical intermediate 25 , which featured two quaternary carbon centres at its bridgehead carbons ( Fig. 7 ). Compound 26 was treated with [RhCl(CO) 2 ] 2 (5 mol%) at 85 °C under an atmosphere of CO (balloon) in ClCH 2 CH 2 Cl. Pleasingly, this reaction proceeded with excellent diastereoselectivity to give the desired product 25 in 86% yield. Subsequent treatment of 25 with NaBH 4 gave lactone 24 in 89% yield, which was subjected to a SeO 2 -mediated allylic oxidation in 1,4-dioxane at 110 °C to give the allylic alcohol 35 in 65% yield as a single diastereoisomer. The excellent diastereoselectivity observed in this reaction was attributed to the steric bulk over the top face of substrate 24 , which would direct the SeO 2 to approach the double bond from its bottom face (see the 3D structure of 24 in Fig. 7 ). Compound 35 was then subjected to a Pd-catalysed hydrogenation reaction to give product 36 in 95% yield. The stereochemistry of 36 as depicted in Scheme 5 was determined by rotating-frame overhauser effect spectroscopy experiments. Furthermore, nuclear overhauser effect (NOE) experiments revealed a correlation between the H-6′, Ha-4′ and H-6′ protons. 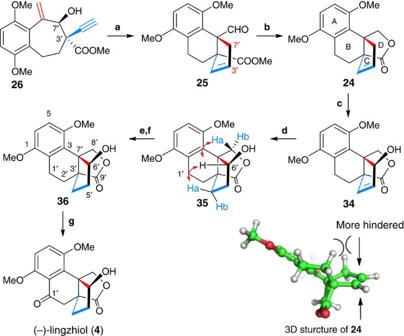Figure 7: Total synthesis of (−)-lingzhiol. (a) [Rh(CO)2Cl]2(5 mol%), CO, DCE, 85 °C, 86%; (b) NaBH4, MeOH, 0 °C, 89%; (c) SeO2, 1,4-dioxone, 110 °C, 65%; (d) Pd-C (10%), H2, MeOH, 25 °C, 95%; (e)N-bromosuccinimide, benzoyl peroxide (BPO), NaHCO3, H2O, CCl4, 80 °C; (f) MnO2, CH2Cl2, 25 °C, 71% for two steps; (g)tBuSH, AlCl3, DCM, 40 °C, 71%. Figure 7: Total synthesis of (−)-lingzhiol. ( a ) [Rh(CO) 2 Cl] 2 (5 mol%), CO, DCE, 85 °C, 86%; ( b ) NaBH 4 , MeOH, 0 °C, 89%; ( c ) SeO 2 , 1,4-dioxone, 110 °C, 65%; ( d ) Pd-C (10%), H 2 , MeOH, 25 °C, 95%; ( e ) N -bromosuccinimide, benzoyl peroxide (BPO), NaHCO 3 , H 2 O, CCl 4 , 80 °C; ( f ) MnO 2 , CH 2 Cl 2 , 25 °C, 71% for two steps; ( g ) t BuSH, AlCl 3 , DCM, 40 °C, 71%. Full size image With the entire lingzhiol skeleton installed, all that remained was to introduce the final oxygen atom at C1′ of 36 and remove its two methoxyl groups. Unfortunately, however, none of the typical benzylic oxidation reaction conditions tested resulted in the desired product 37 . Given that the benzylic position could readily undergo a radical-mediated halogenation reaction, we designed a stepwise protocol involving sequential halogenation/substitution/oxidation reactions to achieve this transformation. Following a period of experimentation, it was established that substrate 36 could be effectively converted to ketone 37 in 73% yield by the sequential treatment of 36 with N -bromosuccinimide (NBS) in the presence of benzoyl peroxide [68] , as well as a trace amount of water in carbon tetrachloride, followed by MnO 2 -mediated oxidation of the resultant benzylic alcohol in CH 2 Cl 2 at room temperature. Finally, removal of the both methoxyl groups of 37 with AlCl 3 in the presence of an excess of t BuSH in CH 2 Cl 2 resulted in the formation of (−)-lingzhiol in 78% yield. The spectroscopic data for the synthetic (−)-lingzhiols were identical to the published values of the natural products [4] and the optical rotation for (−)-lingzhiol ( 4 ) was in good agreement with the literature values ( Supplementary Tables 3–5 ). In summary, we have developed a new intramolecular [3+2] cycloaddition reaction between an enal and an alleno rhodium, which was generated in situ from the Rh(I)-mediated retro-propargylation of the corresponding homo-propargyl alcohol, to give [3.3.0] and [4.3.0] bicyclic ring systems with two quaternary carbon centres at their bridgehead positions. This reaction also allowed for the asymmetric synthesis when it was applied to chiral starting materials. To account for the observed reaction, we proposed a mechanism, which suggested that the reaction might involve an Rh-catalysed ring opening of a 2-alkynyl cycloalkanol moiety followed by the intramolecular [3+2] cycloaddition on an alleno rhodium species to an enal. The application of this reaction to the synthesis of the natural product (−)-lingzhiol has been also achieved for the first time in 17 steps from a commercially available starting material. General For 1 H and 13 C spectra of the compounds in this article, see Supplementary Figs 1–69 . For ORTEP diagrams, see Supplementary Figs 70–76 . For HPLC traces, see Supplementary Figs 77–79 . General procedure for the synthesis of 8 b– 19 b To a solution of an enynol in anhydrous ClCH 2 CH 2 Cl (0.025 M) was added [RhCl(CO) 2 ] 2 (0.5 mg, 1.25 μmol, 5% mol) at CO atmosphere at room temperature and the mixture was degassed with CO for five times. The reaction mixture was then stirred at 85 °C for the time listed in the Tables 2 and 3 . After cooling to room temperature, the solvent was removed under vacuum and the residue was purified by a flash chromatography on silica gel to provide the desired product. For additional procedures, see Supplementary Methods . How to cite this article: Long, R. et al. Asymmetric total synthesis of (−)-lingzhiol via a Rh-catalysed [3+2] cycloaddition. Nat. Commun. 5:5707 doi: 10.1038/ncomms6707 (2014). Accession codes: The X-ray crystallographic coordinates for structures reported in this article have been deposited at the Cambridge Crystallographic Data Centre (CCDC), under deposition numbers CCDC 1026082–1026089. These data can be obtained free of charge from the Cambridge Crystallographic Data Centre via http://www.ccdc.cam.ac.uk/data_request/cif